Observations from old forests underestimate climate change effects on tree mortality Understanding climate change-associated tree mortality is central to linking climate change impacts and forest structure and function. However, whether temporal increases in tree mortality are attributed to climate change or stand developmental processes remains uncertain. Furthermore, interpreting the climate change-associated tree mortality estimated from old forests for regional forests rests on an un-tested assumption that the effects of climate change are the same for young and old forests. Here we disentangle the effects of climate change and stand developmental processes on tree mortality. We show that both climate change and forest development processes influence temporal mortality increases, climate change-associated increases are significantly higher in young than old forests, and higher increases in younger forests are a result of their higher sensitivity to regional warming and drought. We anticipate our analysis to be a starting point for more comprehensive examinations of how forest ecosystems might respond to climate change. Observational studies have relied on old forests to quantify temporal trends in background tree mortality, and have shown that tree mortality has increased with recent global warming, increasing atmospheric CO 2 and decreasing water availability in tropical, temperate and boreal forests [1] , [2] , [3] , [4] , [5] . Old forests are assumed to be in an equilibrium state where tree mortality is matched by recruitment, and temporal changes in tree mortality at the forest level due to endogenous processes are assumed to be weak at this stage of stand development [6] , [7] . However, whether there is ever equilibrium is a contentious issue [8] . Although the effects of competition estimated by temporal changes of stand basal area (SBA) and stand density on tree mortality have been investigated in some previous studies [4] , [5] , conspecific negative density dependence and tree aging could also influence tree dynamics [9] , [10] . Furthermore, the temporal increase of tree mortality could be driven by stand development processes, but not necessarily climate change [11] , [12] . Unfortunately, previous studies have used unsuitable statistical methods that marginalize either climate or non-climate drivers for longitudinal data in which these drivers are highly correlated [13] . Therefore, the relative roles that climate change and stand development processes have on the temporal changes in tree mortality remain uncertain. Furthermore, climate change-associated tree mortality increases in old forests have been used to represent the tree mortality response of regional forests to climate change [14] , based on the assumption that effects of climate change on tree mortality are same for young and old forests. However, this assumption has not been specifically tested. Verification of the assumption is essential for disturbance-driven ecosystems such as boreal forests. Because of high fire frequency, the boreal forests are a mosaic of stands at various developmental stages with old forests accounting for only a small portion of the landscape [15] , [16] . With a predicted increase of fire frequency associated with global warming, the mean age of the boreal forests is expected to decrease, as will the portion of old forests [17] . Thus, understanding how young forests respond to climate change is essential to predict how boreal forests will respond to future climate change. If tree mortality responses to climate change differ between young and old forests, increased tree mortality based on old forests will be biased for regional forest predictions. Here we analyzed tree mortality patterns of boreal tree species in western Canada using 887 permanent sample plots measured between 1958 and 2007. To account for uncertainties in sampling, models and parameters, we used Bayesian models [18] , [19] to disentangle endogenous (stand development) and exogenous (year, temperature anomaly or drought) effects on individual tree mortality for five major boreal tree species, Populus tremuloides Michx., Populus balsamifera L., Pinus banksiana Lamb., Picea mariana Mill. and Picea glauca (Moench) Voss. We tested the assumption that tree mortality increases associated with climate change do not differ with forest age. We also examined whether tree mortality increases are linked to recent regional warming and its negative consequence on water availability. We show that both climate change and forest development processes influence temporal mortality increases, climate change-associated increases are significantly higher in young than old forests, and higher increases in younger forests are a result of their higher sensitivity to regional warming and drought. Furthermore, climate change-associated mortality increases are stronger for moist-habitat-adapted Populus balsamifera and late-successional Picea mariana and Picea glauca than Populus tremuloides and Pinus banksiana. 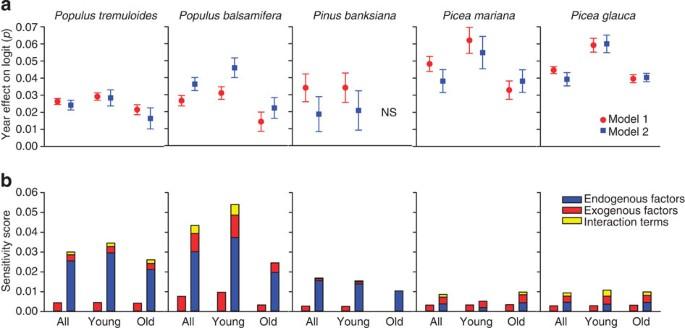Figure 1: Year effect on annual tree mortality probability and sensitivity scores of predictors. (a) Year effect on annual tree mortality probability, logit (p), estimated by Model 1 (without endogenous factors as predictors) and Model 2 (with endogenous factors as predictors). Models were separately developed all plots (All), young plots (Young, initial SA ≤80 years) and old plots (Old, initial SA >80 years), respectively. Error bars are 95% credible intervals. (b) Sensitivity scores. For each species and age group (All, Young or Old), sensitivity scores of predictors from Model 1 are on the left and Model 2 on the right. Effects of year and stand development processes on tree mortality With all data pooled, the effects of year, used to represent climate change drivers as a whole in both Model 1 (with only year as a predictor) and Model 2 (with year, endogenous processes and their interactions as predictors) were significantly positive for all study species ( Table 1 ; Fig. 1 ), indicating significant increases of annual mortality probability during the study period ( Fig. 2 ). The two models, however, produced different estimates for climate change-associated tree mortality: year effects estimated by Model 1 are bigger for Populus tremuloides , Pinus banksiana , Picea mariana and Picea glauca , but smaller for Populus balsamifera than those by Model 2 ( Fig. 1a ), resulting in different estimates of annual tree mortality probability from the two models ( Fig. 2 ). Table 1 Effect of year and its interactive effects with stand development processes on annual mortality probability. Full size table Figure 1: Year effect on annual tree mortality probability and sensitivity scores of predictors. ( a ) Year effect on annual tree mortality probability, logit ( p ), estimated by Model 1 (without endogenous factors as predictors) and Model 2 (with endogenous factors as predictors). Models were separately developed all plots (All), young plots (Young, initial SA ≤80 years) and old plots (Old, initial SA >80 years), respectively. Error bars are 95% credible intervals. ( b ) Sensitivity scores. For each species and age group (All, Young or Old), sensitivity scores of predictors from Model 1 are on the left and Model 2 on the right. 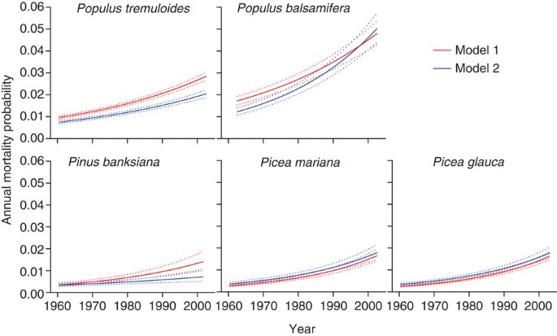Figure 2: Predicted temporal trends of annual mortality probability associated with calendar year. The predicted means (solid lines) and their 95% credible intervals (dotted lines) of annual mortality probability are derived by using equation exp(β)−1, in whichβis the fitted year coefficient from Model 1 (red) and Model 2 (blue) for each respective species inTable 1. Full size image Figure 2: Predicted temporal trends of annual mortality probability associated with calendar year. The predicted means (solid lines) and their 95% credible intervals (dotted lines) of annual mortality probability are derived by using equation exp( β )−1, in which β is the fitted year coefficient from Model 1 (red) and Model 2 (blue) for each respective species in Table 1 . Full size image Tree mortality was strongly affected by stand development processes and their interactions with year ( Fig. 1b , Supplementary Table S4 ). Year effect decreased significantly with stand age (SA) for all study species ( Table 1 ). Year effect also increased with stand crowding as measured by SBA and in stands with more conspecific individuals for Picea mariana and Picea glauca ( Table 1 ). Tree mortality increases associated with year differed among species with stronger year effects on late-successional Picea mariana and Picea glauca and moist-habitat-adapted Populus balsamifera than Populus tremuloides and Pinus banksiana ( Fig. 1a ). When data were analyzed separately for young forests (initial SA ≤80 years) and old forests (initial SA >80 years, same as in Peng et al. [5] ), year effect was consistently higher in young forests than old forests for all species ( Fig. 1a ), supporting the strong declining year effect with increasing SA ( Table 1 ). Predicted annual mortality increased by 2.88%, 4.70%, 5.64% and 6.18% per year in young forests, but increased at the lower rates of 1.65%, 2.24%, 3.89% and 4.12% in old forests for Populus tremuloides , Populus balsamifera , Picea mariana and Picea glauca , respectively ( Supplementary Fig. S3 ). For drought-tolerant Pinus banksiana , annual mortality increased by 2.09% per year in young forests, but year had no detectable effect on its mortality in old forests ( Supplementary Fig. S3 ). In both young and old forests, endogenous factors were critical drivers of tree mortality for all study species ( Fig. 1b ; Supplementary Tables S6 and S7 ). Warming and drought effects on tree mortality For the study area, annual temperature anomaly (ATA) increased at 0.034 °C year −1 , and annual climate moisture index anomaly (ACMIA) decreased at 0.088 year −1 , whereas the growing season precipitation anomaly slightly increased at 0.761 mm year −1 between 1958 and 2007 ( Supplementary Fig. S4 ; Supplementary Table S7 ). To examine whether increase of mortality could be attributed to regional warming and drought, we developed models that replaced year by these climatic variables (Models 3 and 4). The ATA models showed positive main ATA effects on mortality of all species and higher ATA effects in young than old forests of all species except Pinus banksiana ( Table 2 ). The ACMIA models indicated negative main ACMIA effects on mortality of all species and greater effects for Populus balsamifera , Picea mariana and Picea glauca than the other two species. Furthermore, the ACMIA effects were stronger in young than old forests for all species except Pinus banksiana ( Table 2 ). Table 2 Effect of ATA or ACMIA and its interactive effects with stand development processes on annual mortality probability. Full size table Unlike previous attributions of temporal increases in tree mortality to either climate change [1] , [2] , [3] , [4] , [5] or stand development processes [10] , [12] , by using Bayesian models, we show that both stand development processes and climate change have affected temporal increases in tree mortality. These findings are not likely a result of methodological problems because heterogeneity in sampling strategies had no effect on mortality ( Supplementary Figs S5 and S6 ), though we note that we have not explicitly considered alternate exogenous factors here. Tree mortality associated with year decreased for all species except Populus balsamifera when stand development factors were included as predictors. The differences in year effect between the models provide support for the notion that studies excluding endogenous factors can potentially produce biased estimates of climate change effects in boreal forests [13] . The decreased year effect on tree mortality is attributable to stand development processes during the study period. For example, both SA and SBA increased ( Supplementary Table S10 ), both of which positively affected tree mortality ( Supplementary Table S4 ). Also, an increase in the conspecific density of shade-tolerant Picea mariana and Picea glauca ( Supplementary Table S10 ), reflecting the nature of secondary succession in boreal forests [6] , [20] , intensified a negative density-dependence effect on these two species ( Table 1 ). The increased year effect in moist-habitat-adapted Populus balsamifera suggests that reduced water availability might have overweighed endogenous effects. Our results show that mortality increases associated with climate change were significantly higher in young than old forests, and the higher increase in younger forests appears to be due to higher mortality sensitivity to recent regional warming and the resulting negative consequence on water availability. This finding indicates that climate change-associated increases in tree mortality would be underestimated if only old forests are used to represent regional forests. Compared with old forests, even-aged young forests established after a stand-replacing disturbance may experience greater competition for space and nutrients among young trees that tend to occupy the same ecological niche [6] , [7] , resulting in them being more vulnerable to external stressors such as climate change-associated drought [21] , [22] . The positive effect of regional warming on mortality could also be attributed to the interdependencies among warming, drought and forest pests [23] , [24] , [25] . In our study area, outbreaks of forest pests could have a role in the temporal mortality increases [26] , [27] , [28] . Mortality responses to climate change differed among species, suggesting that the regional forest may be undergoing forest compositional shift that is independent of endogenous forest succession. The highest mortality increase in Populus balsamifera among pioneer species indicates that reduced water availability by regional warming has the greatest influence on species adapted to moist habitats. The higher mortality increases of late-successional Picea mariana and Picea glauca than those of early-successional Populus tremuloides and Pinus banksiana in both young and old forests ( Figs 1 and 2 ) suggest that the regional forest will likely become further dominated by early-successional species if current warming trends continue. The different responses of tree mortality among species, coupled with those by climate change-associated fire activities [15] , [16] , [17] , [29] that promote early-successional species [30] , may pose a significant conservation challenge for the region under further global warming. We show evidence that long-term tree mortality trends are influenced by both stand development processes and long-term climate trends, that is, regional warming and drought. Note that the strength of these drivers on tree mortality differs among species, and their influences interact both among endogenous factors and between endogenous and exogenous factors. Because of the higher sensitivity to recent climate change in young than old forests, climate change-associated tree mortality could be underestimated if mortality estimates from old forests are used to represent regional forests. Tree mortality responses to climate change differed among species, and these different responses can have strong implications for future forest composition in the western boreal forest. Study area and the forest inventory data We analyzed longitudinal data from 887 permanent sampling plots established in Alberta and Saskatchewan ( Supplementary Data 1 and Supplementary Fig. S1 ). Details for plot establishment, measurements and selection criteria are described in Supplementary Methods . Explanatory variables To examine whether long-term tree mortality trends are affected by long-term climate change trends, similar to previous studies [1] , [2] , [3] , [4] , [5] , [12] , we used the middle calendar year of a census period, during which tree mortality measurements were made between two successive censuses, to represent climate change drivers as a whole. To account for the effects of endogenous factors including asymmetric competition, stand crowding, tree ageing and inter-specific interaction on tree mortality, we used the tree’s relative basal area (RBA; ratio of subject tree basal area to the mean tree basal area of the stand), SBA, SA and the ratio of focal species’ basal area to SBA, calculated using the preceding measurement of each census period [10] . Climate anomalies were defined as the departure from the long-term climate means [31] . Because our dependent variable, tree status, was observed at the end of a census period, the departure from the long-term mean for each climate variable was defined as the difference between its mean value during the census period and its long-term mean. Long-term climate means were calculated based on the 1950–2007 time period, during which plot measurements were taken. Three sets of climate anomalies were calculated: ATA, growing season precipitation anomaly and ACMIA. We derived temperature and precipitation data using scale-free ClimateWNA [32] , [33] and climate moisture index (CMI) using BioSIM [34] from latitude, longitude and elevation of each sample plot. Annual CMI was the sum of monthly CMIs over 12-month periods from last 1 August to 31 July of the current year, where monthly CMI was the quantity of monthly precipitation minus monthly potential evapotranspiration, which was computed using a simplified form of the Penman–Monteith equation [35] . A smaller CMI value indicated a drier condition. The summary statistics for explanatory variables were presented in Supplementary Table S2 . Annual mortality probability calculations We used individual tree mortality analyses rather than plot-level mortality analyses to accommodate the individual tree-level variable, RBA, because (1) RBA is the strongest predictor of tree mortality in non-equilibrium boreal forests and (2) its control on tree mortality can change with SBA and ratio of focal species’ basal area to SBA [10] . Similar to previous studies [36] , [37] , we were interested in estimating annual tree mortality probability where measurement intervals varied ( Supplementary Fig. S2e ). We derived annual mortality probability from tree status as follows. The survival probability, S , of tree i , for census period j of t years, in plot k is expressed as a function of annual survival probability, s : Lastly, we related a tree’s status at the end of the census period ( M ijk , alive or dead) to annual mortality probability using Bernoulli likelihood: Statistical analyses For each species, we developed individual tree mortality models using Hierarchical Bayesian logistic regression with plot identity as a random effect to account for uncertainties potentially affected by different forest characteristics or in different climatic and/or edaphic conditions [18] , [19] . where α and β are the intercept and estimated coefficients, respectively; X ijk represents explanatory variables corresponding to tree i for census period j in plot k ; and the model included a term π k to describe the random effect of sampling plots. As a rule of thumb, π k is in normal distribution with a mean of 0. To examine whether inclusion of endogenous factors alters climate change-associated tree mortality, we compared the year effect between models with and without inclusion of endogenous factors as predictors, that is, Model 1 and Model 2, respectively. where f ( En ) in Model 2 was developed based on our previous work [10] to account for the endogenous effects on tree mortality: where β s are the coefficients. We modelled the mortality probability as an exponential function of RBA because our previous results showed that mortality probability decreases exponentially with RBA [10] . The Akaike information criterion also indicated that the exponential transformation of RBA gave better fits for all species ( Supplementary Table S3 ). Furthermore, our previous work [10] showed near-linear mortality trends with tree aging and with SBA after taking account of competition and species interaction. Consequently, we modelled mortality probability as a linear function of SA and SBA. Both Models 1 and 2 were developed for all plots, young forest plots and old forest plots, respectively, to examine how the inclusion of endogenous factors affect year effect in these three scenarios. Following Peng et al. [5] , we defined that young forests were ≤80 years of age and old forests >80 years of age at the first census. To examine whether increases of mortality could be attributed to regional warming and its negative consequence on water availability, we developed models that replaced year with the climatic variables in Model 2, resulting in Models 3 and 4. To examine the temporal trends of endogenous and exogenous factors at the plot level, Y, we used the Hierarchical Bayesian linear (HBL) model. where Y jk is dependent variable, that is, endogenous factors and exogenous factors; α and β are intercept and estimated coefficients, respectively; Year jk represents middle calendar year at for census period j in plot k ; and the model included a term π k to describe the random effect of sampling plots. For all analyses, the Bayesian Markov Chain Monte Carlo methods were implemented using JAGS [38] called from R [39] with rjags package [40] . All coefficients were assigned non-informative priors. All independent variables were centred to reduce their correlations and speed up convergence. For each model, we evaluated convergence by running two independent chains with different initial values and monitoring the Gelman–Rubin statistic [41] . When convergence was confirmed, an additional 10,000 iterations with thinning of half were used to calculate the mean, s.d. and 95% credible interval for each coefficient from the posterior distribution. We developed full models and sequentially removed dimensionless explanatory variables whose posterior 95% credible interval covered 0. The reduced models, assessed by Deviance Information Criterion, were better than or similar to full models ( Supplementary Table S11 ). Consequently, we selected the reduced models as our final models. To assess the adequacy of the final models, we calculated the area under the receiver operating characteristic curve (AUC) based on the mean of each coefficient using ROCR package [42] . A value of AUC >0.8 indicates that a model has excellent discriminatory power, and a value >0.7 indicates good discriminatory power [43] . Finally, we calculated the mortality sensitivity scores to endogenous factors, exogenous factors and their interactions as a measure of the influences of these factors on mortality. Similar to Dietze and Moorcroft [37] , we defined sensitivity score on annual mortality probability as the s.d. of the predicted annual mortality probability for each of the above three groups of factors, holding the other two groups of variables at their mean. To present how annual mortality probability changes over the study period, we summarized posterior distribution of annual mortality probability (mean and 95% credible interval) using mean of each parameter ( β ) from the final models. We also calculated the annual fractional change of mortality probability associated with year over the study period using the equation exp( β )−1, in which β is fitted coefficient for Year. Assessing possible methodological problems We first examined the spatial auto-correlation and heterogeneity in sampling strategies following the method described by van Mantgem et al. [4] . For all study species, Mantel tests showed no evidence of spatial auto-correlation among the plots for annual mortality probability, annual fractional change of mortality probability or the effect of plot identity on annual mortality probability ( Supplementary Table S12 ). The selected permanent sampling plots were located in ecologically heterogeneous regions, and close geographic configuration does not imply similarity in forest characteristics. Our result that mortality probability increased more so in young forests than old forests could also be mistaken if the young forest plots were spatially clustered. Thus, we also examined the spatial auto-correlation for initial SAs. For all study species, the mantel tests showed no evidence of spatial auto-correlation among the plots for initial SA ( Supplementary Table S12 ). The linear regressions that related annual mortality fractional change to plot size and average census interval showed that neither plot size nor average census interval was significantly related to annual mortality fractional change ( Supplementary Figs S5 and S6 ). These results indicate that the variation of mortality changes could not be attributed to plot size heterogeneity or the variation in census intervals. How to cite this article: Luo, Y. and Chen, H.Y.H. Observations from old forests underestimate climate change effects on tree mortality. Nat. Commun. 4:1655 doi: 10.1038/ncomms2681 (2013).